Non-invasive classification of microcalcifications with phase-contrast X-ray mammography Microcalcifications can be indicative in the diagnosis of early breast cancer. Here we report a non-invasive diagnostic method that may potentially distinguish between different types of microcalcifications using X-ray phase-contrast imaging. Our approach exploits the complementary nature of the absorption and small-angle scattering signals of microcalcifications, obtained simultaneously with an X-ray grating interferometer on a conventional X-ray tube. We demonstrate that the new approach has 100% sensitivity and specificity when applied to phantom data, and we provide evidence of the solidity of the technique by showing its discrimination power when applied to fixed biopsies, to non-fixed tissue specimens and to fresh, whole-breast samples. The proposed method might be further developed to improve early breast cancer diagnosis and has the potential to increase the diagnostic accuracy and reduce the number of uncomfortable breast biopsies, or, in case of widespread microcalcifications, to select the biopsy site before intervention. Absorption-based X-ray mammography, in combination with ultrasonography, is the actual standard in breast cancer detection [1] , [2] . The identification of (clustered) microcalcifications is one goal of breast cancer screening and early detection of pre-malignant and malignant lesions. Breast calcifications are common on mammograms being especially prevalent after menopause. Although they are usually benign, certain morphologic (for example, fine pleomorphic or fine linear) and distribution (for example, clustered or segmental distribution) descriptors may indicate breast cancer [3] . The non-invasive discrimination of type I and type II microcalcifications, see below, could provide an additional descriptor for a scoring system to stratify the risk of malignancy or pre-malignancy within present clusters of microcalcifications [4] . In patients who present with several clusters of microcalcifications, for example, in suspected sclerosing adenosis, and have been scheduled for vacuum-assisted biopsy, this may further help in selecting the best area for intervention [5] . Microcalcifications consist of tiny calcium deposits that may be present in areas of accelerated cell turnover, indicative for pre-cancerous changes or early invasive breast cancer. In the clinical routine, areas with suspicious microcalcifications within a breast are further investigated by stereotactic vacuum biopsies, followed by the histopathological workup. Frappart et al. [6] , [7] have introduced the existence of two types of microcalcifications of different chemical composition as well as their correlation with benign and malignant breast lesions [6] , [7] , [8] . Type I microcalcifications consist of calcium oxalate dihydrate while type II microcalcifications are composed of calcium phosphates, mainly calcium hydroxyapatite [9] . Type I microcalcifications are seen most frequently in benign ductal lesions and are rarely associated with breast cancer. Type II microcalcifications are found in both benign and malignant lesions, but are most often found in proliferative lesions, including invasive breast cancer [8] , [9] , [10] . Invasive and non-invasive investigations can be carried out to discern these two types of microcalcifications. Non-invasive methods rely on conventional absorption-based mammography, attempting to correlate morphological parameters such as the shape, size, number and roughness of the detected microcalcifications [11] , [12] , [13] . The underlying algorithms bear limitations such as a dark background, densely clustered calcifications or low-density calcific flecks [9] . Moreover, the morphological information is not specific and therefore such algorithms are limited to specific cases and mammograms, and are found not to be reliable for this purpose. Invasive methods are more rigorous, including near-infrared Raman spectroscopy [9] (rather unpractical in a clinical environment owing to its experimental complexity and poor throughput) and histopathology, the standard in the clinical routine. Raman spectroscopy is chemical specific, and therefore well suited to determine different types of microcalcifications, but it works only on very thin, sliced tissue samples, obtained invasively with a biopsy, owing to the very limited penetration power of the probing radiation. In histopathology, using haematoxylin and eosin staining, the two types of microcalcifications show different refractive properties (type I is found to be birefringent, while type II is non-birefringent [6] , [7] , [9] ) when polarized light is used thus allowing their discrimination. Phase-contrast X-ray imaging has the potential to significantly improve the radiographic accuracy of mammographic investigations [14] , [15] , [16] . Recently, using an X-ray Talbot–Lau grating interferometry (GI) [17] , [18] , we generated phase-contrast mammograms of non-fixed human whole-breasts samples ex vivo [19] , [20] . Our imaging technique records absorption, differential phase and small-angle scattering signals from the sample simultaneously [18] , [21] . Especially for breast diagnostics, the GI technique may provide superior contrast compared with conventional absorption-based X-ray imaging, and might potentially reduce dose deposition to the sample [19] . In this paper, we present a method based on GI, which may non-invasively distinguish between type I and type II microcalcifications. The method relies on the observation that the aforementioned two types of microcalcifications show opposite absorption and small-angle scattering signals. Compared with conventional mammography, our approach reflects the internal crystal structure of the microcalcifications in addition to the morphological information. Grating interferometer setup with X-ray tube configuration The layout of the grating interferometer is sketched in Fig. 1 . Together with a conventional X-ray tube source (generating a continuous Bremsstrahlung spectrum) and an area detector, which are the standard components in conventional radiography, three X-ray gratings (G0, G1 and G2) [18] are arranged at predefined positions between the source and detector [17] , [18] . 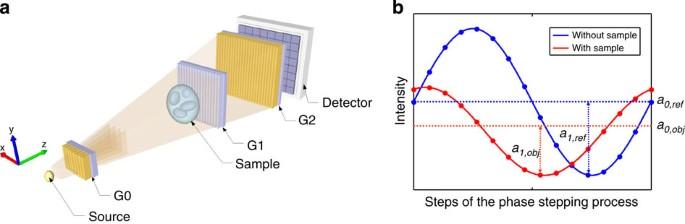Figure 1: The scheme of a grating interferometer. (a) The phase grating G1 generates an interference pattern at the position of the analyser grating G2. A sample in front of the phase grating causes a distortion of the interference pattern. G2 is used to analyse the interference pattern and obtain information about the sample. (b) For each pixel of the detector, two phase-stepping curves, one without sample (blue) and one with the sample (red), are obtained. From those curves, the absorption, differential phase and scattering signals are retrieved. Figure 1: The scheme of a grating interferometer. ( a ) The phase grating G1 generates an interference pattern at the position of the analyser grating G2. A sample in front of the phase grating causes a distortion of the interference pattern. G2 is used to analyse the interference pattern and obtain information about the sample. ( b ) For each pixel of the detector, two phase-stepping curves, one without sample (blue) and one with the sample (red), are obtained. From those curves, the absorption, differential phase and scattering signals are retrieved. Full size image The phase grating G1, whose lines are typically made of silicon and periodically introduce a phase shift of zero and π to the X-ray wavefront, works as a beam splitter. The periodic phase modulation generates, due to wave interference, a periodical intensity distribution downstream of G1, which appears as fringes perpendicular to the beam direction. To generate the interference pattern, the source needs to be sufficiently coherent, which is not the case for commercially available mammography X-ray tubes, showing typically a focal spot size of hundreds of microns. Therefore, an absorption (with gold lines) grating G0 has to be placed immediately after the source, effectively splitting the source into an array of micron-sized sources, yielding the required partial coherent illumination of the sample [18] . The sample on the beam path, distorts the interference pattern downstream G1 due to the attenuation, refraction and scattering of the X-rays when passing through the specimen. To obtain and separate these signals, an analyser grating G2 (absorption grating with gold lines) with the same periodicity as the fringes is placed downstream G1, exactly at the location of such fringes, known as the Talbot or Lohmann distance [22] . G2 acts as a mask, which encodes the mean fringe shift within a detector pixel into an intensity value. During the data acquisition, one of the gratings is moved transversally step-by-step following the so-called phase-stepping process [18] , [23] . For each pixel on the detector, two pseudo-sinusoidal intensity curves (phase-stepping curves) with/without sample are obtained ( Fig. 1b ). In this work, we focus on the absorption and the small-angle scattering signals, T and S , respectively, which are defined as: where a i is the magnitude of the i -th Fourier component of the phase-stepping curve, and are defined as the visibilities of the phase-stepping curves, with and without an object, respectively [21] . In classical radiography, the minus logarithm of the absorption signal T is well known as the line integral of the attenuation coefficients, and the minus logarithm of the scattering signal S is directly proportional to the linear integration of the generalized scattering parameters [24] : where L is the thickness of the specimen, μ is the attenuation coefficient, s is the generalized scattering parameter and c is a constant depending on the geometry and system parameters of the grating interferometer. Non-invasive microcalcifications classification The difficulty of distinguishing two types of microcalcifications with conventional mammography is twofold. First, current absorption-based mammography yields only morphological information on the microcalcifications while it lacks in providing hints about their chemical composition and structure. Second, conventional mammography bears the two-dimensional limitation, namely that the thickness of a microcalcification cannot be determined from the mammograms. Therefore, although two types of microcalcification may have different attenuation coefficients, they still cannot be classified owing to their unknown thickness. X-ray GI solves these two flaws simultaneously. By considering the small-angle scattering signal as complementary to the absorption signal, our method can analyse the differences in the attenuation coefficient as well as in the crystal structure of the microcalcifications, and uses the scattering signal to decouple the thickness parameter. The method relies on our first observations that type I and type II microcalcifications yield opposite absorption and scattering signals. For a given microcalcification thickness, one type gives a weaker absorption signal but a stronger small-angle scattering signal than the other type, and vice versa. Since there are only two kinds of microcalcifications and their absorption and small-angle scattering signals are opposite, we can uniquely determine their types by exploiting this correlation. Suppose there are two microcalcifications ( A and B ), which give opposite absorption and scattering signals. Without loss of generality, we suppose T l,A < T l,B and S l,A > S l,B , where T l represents the absorption signal and S l represents the small-angle scattering signal (equations (2) and (3)). If T l,A < T l,B , there are two possible reasons: either they are the same type (having the same attenuation coefficients), but the thickness of B is larger than A or they have different attenuation coefficients, representing different types of microcalcifications. This ambiguity can be removed by exploiting the small-angle scattering signals. If it is the former case, we will get L A < L B where L represents the thickness. According to the linear relationship of the small-angle scattering power with the thickness, S l,A > S l,B is not allowed, yet belong to different types of microcalcifications. To decouple the thickness parameter, the ratio of equation (3) to equation (2) (or vice versa) can be used [25] , which is The two types of microcalcifications can be separated with a threshold t , The threshold is obtained from the statistical analysis of a large number of known microcalcifications and it ultimately defines the sensitivity and specificity of the method. Validation of phantom data In a preliminary step, we validated our findings by designing a phantom using simulants mimicking the main chemical composition of the type I and type II microcalcifications. The simulants have been chosen according to the work of Haka et al. [9] who demonstrated by Raman spectroscopy that calcium oxalate dihydrate (CaC 2 O 4 ·2H 2 O) and calcium hydroxyapatite (Ca 5 (PO 4 ) 3 (OH)) are the major components of type I and type II microcalcification, respectively. Besides their difference in X-ray attenuation coefficient, these two types of materials present different crystal properties. The results are shown in Fig. 2 . The two materials behave as expected, showing opposite absorption and scattering signals. Our experimental observations indicate that type I microcalcifications generally show a smaller attenuation signal compared with type II microcalcifications. Further, type I microcalcifications are reported to be made of monocrystals or are associations of monocrystals (observed as pyramids or dipyramids of crystallines in scanning electron microscopy) [7] , and are therefore expected to induce stronger refraction to X-rays passing through them. This behaviour affects the small-angle scattering signal recorded with GI [18] and, as a consequence, it becomes detectable. On the contrary, type II microcalcifications are found to be non-crystalline. Therefore, for the same thickness, type I microcalcifications are expected to give a higher scattering signal than type II microcalcifications. 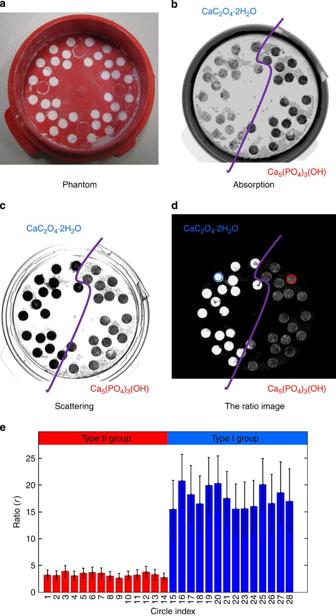Figure 2: Qualitative validation using microcalcification simulants. (a) Phantom designed to simulate different types of calcifications. (b) The absorption image of the phantom. The two types of calcifications show different X-ray absorption properties. (c) The small-angle scattering image of the phantom. The scattering signals are opposite to the absorption signals. (d) The ratio signal shows a clear discrimination between the two microcalcifications simulants. (e) The bar plot shows the means of thersignal of the circles in (d). The error bars represent the s.d. of thersignal. Each group contains 14 circles. Figure 2: Qualitative validation using microcalcification simulants. ( a ) Phantom designed to simulate different types of calcifications. ( b ) The absorption image of the phantom. The two types of calcifications show different X-ray absorption properties. ( c ) The small-angle scattering image of the phantom. The scattering signals are opposite to the absorption signals. ( d ) The ratio signal shows a clear discrimination between the two microcalcifications simulants. ( e ) The bar plot shows the means of the r signal of the circles in ( d ). The error bars represent the s.d. of the r signal. Each group contains 14 circles. Full size image For each circular region in the phantom, the mean and standard variance of the r signal (equation (4)) have been calculated and the results are shown in Fig. 2e . A statistically significant, clear discrimination between the two types of microcalcifications is observed, resulting in 100% sensitivity and 100% specificity in microcalcification classification. A two-sample t -test without equal variances assumption (MATLAB and Statistics Toolbox R2013b, The MathWorks Inc., Natick, MA, United States) has been performed and the null hypothesis has been rejected with p <0.001, indicating the two simulants groups can be correctly classified using our method. Classification in fixed tissue We investigated a biopsy breast tissue with severe microcalcifications fixed in 4% formalin solution, see Fig. 3 , where we could identify 238 microcalcifications of size ranging from 100 to 500 μm. Using the ratio signal r in equation (4), the calcifications in Fig. 3a could be classified into two categories as shown in Fig. 3d , presenting different behaviours in the absorption and scattering signals. Additional details are given in the Supplementary Fig. 1 . Microcalcifications presenting opposite absorption and scattering signals are clearly visible ( Fig. 3c ). It is worth mentioning that this phenomenon exists for microcalcifications of various sizes as can be observed in Fig. 3c as well. The two microcalcifications indicated by the yellow arrows for instance, are of similar size but show totally different behaviours of their absorption and scattering signals. The blue group in Fig. 3d is associated with type I microcalcifications while the red group matches type II. For this particular biopsy sample (resected from a malignant breast lesion), the red group contains more (229) microcalcifications than the blue group (9), which is consistent with the observations that type II microcalcifications occur more frequently than type I, and are most likely associated with malignant breast lesions [26] . The same opposite signals phenomenon is also observed in fresh human whole-breast samples (see Supplementary Fig. 2 ). 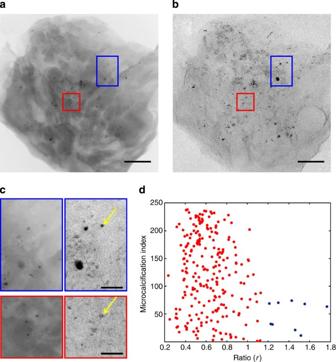Figure 3: Experimental observation of two types of calcifications. A 4% formalin-fixed breast tissue sample investigated with grating interferometry showing two types of microcalcifications with absorption and small-angle scattering signals. (a) Absorption image of the specimen carrying microcalcifications. (b) Corresponding small-angle scattering image of the same specimen. The images show the signals defined in equation (1) in an inversed grey level scale, to give a better visual perception of the microcalcifications. The same colour map is applied for all sample images in this paper. (c) Details of the region of interest (ROI) delineated by the red and blue rectangles shown in (a,b). The microcalcifications within the blue rectangle have weaker absorption signals but stronger scattering signals, while those within the red rectangle have relatively stronger absorption signals but weaker scattering signals. (d) The distribution of all the visible microcalcifications in the specimen with respect to the ratio defined in equation (4). Scale bars, 1 cm in (a,b); 5 mm in (c). Figure 3: Experimental observation of two types of calcifications. A 4% formalin-fixed breast tissue sample investigated with grating interferometry showing two types of microcalcifications with absorption and small-angle scattering signals. ( a ) Absorption image of the specimen carrying microcalcifications. ( b ) Corresponding small-angle scattering image of the same specimen. The images show the signals defined in equation (1) in an inversed grey level scale, to give a better visual perception of the microcalcifications. The same colour map is applied for all sample images in this paper. ( c ) Details of the region of interest (ROI) delineated by the red and blue rectangles shown in ( a , b ). The microcalcifications within the blue rectangle have weaker absorption signals but stronger scattering signals, while those within the red rectangle have relatively stronger absorption signals but weaker scattering signals. ( d ) The distribution of all the visible microcalcifications in the specimen with respect to the ratio defined in equation (4). Scale bars, 1 cm in ( a , b ); 5 mm in ( c ). Full size image Classification in fresh non-fixed tissue biopsy As a next step, we applied our method to a non-fixed sample, obtained from a fresh biopsy, and we validated our results with histopathology. Correlating the microcalcifications identified in the phase-contrast images with the ones selected for the histopathological workup is notably a challenging task. Some microcalcifications detected in the phase-contrast images have been used as ‘fiducials’ to increase the probability of successful identification. 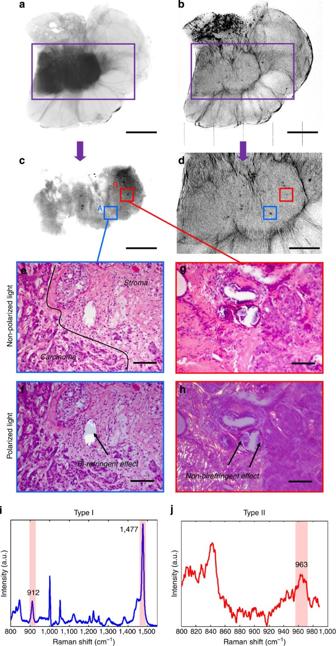Figure 4: Classification in a non-fixed breast cancer tissue sample. Absorption (a) and scattering (b) images of the biopsy sample. (c) Region of interest (ROI) of the absorption image. The display window has been adapted to clearly show the microcalcifications. (d) The scattering image of the same ROI. The type I microcalcification is delineated with blue colour and the type II is marked with red colour. (e,f) are the histological images of type I calcification (around 250 μm) under non-polarized and polarized light, respectively. (g,h) are the histological images of type II calcification (around 400 μm) under non-polarized and polarized light, respectively. (f) shows the birefringent property of the type I microcalcification by the use of polarized light. The type II microcalcification does not exhibit this property in (h). (i,j) are the Raman spectra of the type I and type II microcalcifications, respectively. Scale bars, 1 cm in (a,b); 5 mm in (c,d); 500 μm in (e–h). Figure 4 shows a typical set of absorption and scattering images ( Fig. 4a ; Fig. 4b , respectively) where two microcalcifications have been marked to be the target of the follow-up histological analysis ( Fig. 4c,d ). According to our method, we temporarily label one of them (A) as type I, as it shows lower absorption but higher scattering signals than the other one (B). B is labelled as type II, as it shows opposite behaviour. The corresponding histopathological examinations revealed that A displayed birefringent optical properties, indicating a crystalline structure ( Fig. 4f ): as a consequence, A can be classified as type I microcalcification. The type I microcalcification was found to be located in the stroma adjacent to the carcinoma as shown in Fig. 4e . Microcalcification B, located within a duct surrounded by tumour masses and collagen fibres, shows non-birefringent properties and, therefore can be classified as type II ( Fig. 4g,h ). Histopathology thus confirms the predictions made by our method and supports our hypothesis that this approach may be able to discriminate microcalcification of different types non-invasively. To further verify the chemical compositions of the microcalcifications, we used Raman spectroscopy to identify the main chemical signatures of the two microcalcifications. Their Raman spectrums are shown in Fig. 4i,j , respectively. The spectrum of the type I microcalcification shows the characteristic signature peaks at 912 cm −1 and 1,477 cm −1 , indicating the presence of calcium oxalate dihydrate in crystalline form. The spectrum of the (non-crystalline) type II microcalcification shows the signature peak at ~963 cm −1 , which corresponds to calcium hydroxyapatite. These results are consistent with the measurements of Haka et al. [9] Figure 4: Classification in a non-fixed breast cancer tissue sample. Absorption ( a ) and scattering ( b ) images of the biopsy sample. ( c ) Region of interest (ROI) of the absorption image. The display window has been adapted to clearly show the microcalcifications. ( d ) The scattering image of the same ROI. The type I microcalcification is delineated with blue colour and the type II is marked with red colour. ( e , f ) are the histological images of type I calcification (around 250 μm) under non-polarized and polarized light, respectively. ( g , h ) are the histological images of type II calcification (around 400 μm) under non-polarized and polarized light, respectively. ( f ) shows the birefringent property of the type I microcalcification by the use of polarized light. The type II microcalcification does not exhibit this property in ( h ). ( i , j ) are the Raman spectra of the type I and type II microcalcifications, respectively. Scale bars, 1 cm in ( a , b ); 5 mm in ( c , d ); 500 μm in ( e – h ). Full size image Classification in fresh whole-breast samples As a final step, we applied our method for the classification of microcalcifications in fresh, whole-breast samples obtained from resection. The phase-contrast images have been acquired in the framework of a recent study, approved and carried out at the Kantonsspital Baden, Switzerland [20] . Owing to the sample inclusion criteria of that study, all the mastectomy samples contained invasive carcinoma. Therefore, we expect the occurrences of the type II microcalcifications to be much higher than type I. 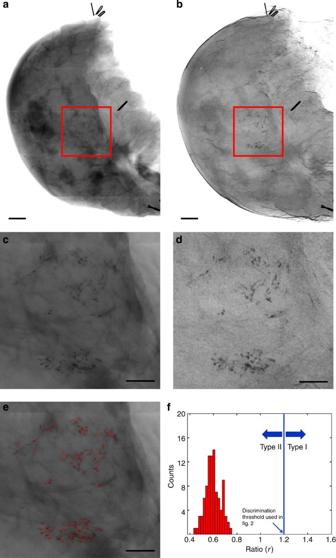Figure 5: Classification results in a non-fixed whole-breast sample. Absorption image (a) and scattering image (b) of the whole breast (compressed thickness of 4.5 cm). (c) Close-up absorption image of the region of interest (ROI) marked in (a); (d) close-up scattering image of the ROI marked in (b); (e) 94 microcalcifications were marked out in the ROI with red circles; (f) shows the histogram of the ratio values of the 94 microcalcifications. The sizes of the observed microcalcifications vary from 100 to 800 μm. The ratio values were normally distributed around a peak value of 0.6, indicating no significant deviations in their ratio values. Scale bars, 2 cm in (a,b); 1 cm in (c–e). Figure 5 shows the classification of microcalcifications detected in a mastectomy sample from a patient with a ductal invasive, hormone receptor and HER-2-neu-positive breast cancer with surrounding high-grade ductal carcinoma in situ . In this particular sample, no opposite absorption and scattering signal effects are observed. Only one type of microcalcification can be identified, as the ratio values for all the microcalcifications are found to be normally distributed in the range of 0.45~0.75 around a peak value of 0.6 as shown in Fig. 5f . Following the same empirical threshold suggested in Fig. 3 all those microcalcifications are classified as type II. We verified our prediction with histopathology, and, as expected, in the region of interest (ROI) region shown in Fig. 5c only non-birefringent type II microcalcifications were found. The microphotographies of two selected microcalcifications are shown in the Supplementary Fig. 3 . Both show non-birefringent properties under polarized light, as typical for type II microcalcifications. Figure 5: Classification results in a non-fixed whole-breast sample. Absorption image ( a ) and scattering image ( b ) of the whole breast (compressed thickness of 4.5 cm). ( c ) Close-up absorption image of the region of interest (ROI) marked in ( a ); ( d ) close-up scattering image of the ROI marked in ( b ); ( e ) 94 microcalcifications were marked out in the ROI with red circles; ( f ) shows the histogram of the ratio values of the 94 microcalcifications. The sizes of the observed microcalcifications vary from 100 to 800 μm. The ratio values were normally distributed around a peak value of 0.6, indicating no significant deviations in their ratio values. Scale bars, 2 cm in ( a , b ); 1 cm in ( c – e ). Full size image We recently showed that many crucial diagnostic aspects such as general image quality, clinical relevance or sharpness and delineation of lesions are significantly superior on phase-contrast mammograms than in images obtained with conventional, absorption-based mammography [20] . This is a strong, statistically supported indication that phase-contrast imaging can play a significant role in breast imaging. In this work, we propose a non-invasive diagnostic method to distinguish between two different types of microcalcifications using X-ray phase-contrast imaging. We show that the two types of microcalcifications can be identified using the opposite behaviour of their absorption and scattering signals obtained with a grating interferometer operated in a simple, radiographic mode. On the basis of the supportive indications presented in ref. 20 , and the evidence presented in this work, namely that our technique can successfully discern between type I and type II microcalcifications in fixed biopsies, fresh tissue and fresh whole-breast samples, we are convinced that this novel approach will improve diagnostic accuracy and ultimately provide a better, early breast cancer detection. The mean glandular dose for a 4.5-cm-thick breast sample is measured to be 26.2 mSv as described in ref. 19 . This high dose is mainly caused by the non-optimal design of the experimental instrument, which is rather a demonstrator than a clinical prototype. With an optimized design of each component, as described in detail in ref. 19 , the dose could be reduced by more than one order of magnitude, matching the European Guidelines [27] while maintaining the same image quality. Further work will involve statistical analysis of a larger number of cases acquired on an improved prototype, with the aim to investigate sensitivity and specificity of the novel approach in a clinical environment. Experimental system and imaging protocol The grating interferometer for mammography is set up at the Paul Scherrer Institut, Villigen, Switzerland. The system uses a Seifert ID 3000 X-ray generator and an unfiltered tungsten line focus tube, which is operated at 40 kVp with a mean energy of 28 keV and a current of 25 mA. The periods of the gratings are 14, 3.5 and 2.0 μm for G0, G1 and G2, respectively. The detector is a Hamamatsu C9732DK flat panel CMOS detector featuring a 12 × 12 cm 2 field of view with 50 × 50 μm 2 pixel size. The distance from the G0 grating to the G1 grating was 140 cm, and from G1 to G2 the distance was 20 cm. The resulting field of view, limited by the size of the G1 and G2 gratings, was 6 × 6 cm 2 . During the data acquisition, 16 steps were used with an exposure time of 7 s (for biopsy) or 9 s (for mastectomy) for each. The Raman spectroscopy measurements were done on a HORIBA Jobin Yvon LabRAM HR800 Raman system equipped with a He-Ne laser (632.8 nm wavelength) measuring in backscattering geometry. A × 50 objective was used to focus the laser beam down to a region of ~2 μm in diameter within the microcalcifications. Sample preparation and histopathological investigation The biopsies are taken from mastectomy samples. The biopsy used in Fig. 3 is a formalin-fixed sample while the other biopsies included in this study are non-fixed tissue samples. The official ‘Institutional Review Board’ (IRB) of the Kantonsspital Baden approved this study and written informed consent was obtained from all patients. Eligible samples contain pre-confirmed microcalcifications or microcalcification clusters identified in in vivo mammograms. Immediately after resection, several 4 × 4 × 1 cm 3 -biopsy samples are taken from a pre-marked region with suspicious microcalcifications. Imaging is performed at the Paul Scherrer Institut within 2 h after resection. Biopsy samples are individually fixed in a dedicated sample holder with adequate compression (around 8 mm thickness) and went through a fast X-ray phase-contrast scan to filter out samples without microcalcifications. The holder is filled with liquid paraffin to avoid strong phase wrapping at the sample-air border. Samples with observable microcalcifications are chosen and scanned with a more sensitive (16 phase steps) phase-contrast procedure. The absorption and scattering images are examined and suspicious microcalcifications are marked in the images according to the proposed method. After X-ray imaging, the tissue samples undergo standard histopathological examination. The whole samples are embedded in paraffin blocks and sliced with 5 μm thickness to form a three-dimensional data set. All slices are then stained (standard haematoxylin and eosin stain) and examined by microscopy with both unpolarized and polarized light to identify the birefringent and non-birefrigent microcalcifications [7] . The types and locations of the found microcalcifications are marked and the histopathological findings are compared with the experimental imaging results. The sample preparation and imaging protocol for mastectomies are similar as those for biopsies. More details can be found in our publications (refs 19 and 20 ). How to cite this article: Wang, Z. et al. Non-invasive classification of microcalcifications with phase-contrast X-ray mammography. Nat. Commun. 5:3797 doi: 10.1038/ncomms4797 (2014).